Multinuclearin situmagnetic resonance imaging of electrochemical double-layer capacitors The last decade has seen an intensified interest in the development and use of electrochemical double-layer capacitors, fuelled by the availability of new electrode materials. The use of nanoporous carbons, in particular, with extremely high surface areas for ion adsorption has enabled the development of working devices with significantly increased capacitances that have become viable alternatives to lithium-ion batteries in certain applications. An understanding of the charge storage mechanism and the ion dynamics inside the nanopores is only just emerging, with the most compelling evidence coming from simulation. Here we present the first in situ magnetic resonance imaging experiments of electrochemical double-layer capacitors. These experiments overcome the limitations of other techniques and give spatially resolved chemical information about the electrolyte ions in real time for a working capacitor of standard geometry. The results provide insight into the predominant capacitive processes occurring at different states of charge and discharge. Advances in electrochemical double-layer capacitors (EDLCs) in recent years [1] , [2] , [3] , [4] have been promoted by the observation of anomalously large capacitances in systems using nanoporous carbon-based electrodes with small pore sizes that are slightly larger than the solvated electrolyte ions [5] , [6] . A number of mechanisms have been proposed to explain the increased capacitance, including the reduction of overscreening effects of the ions in the double layer due to the confinement of ions in small pores [7] , [8] , the screening of the ions in the pores allowing them to come closer together [9] and the stripping of the solvation shell from the ions on their entering the pores. The latter effect results in a closer approach of the molecules to the electrode surface, the process of stripping itself representing a significant energy storage mechanism [6] . These results have driven research into the synthesis of novel carbon materials with a range of properties [10] , [11] and tuneable pore sizes [12] , and also highlight the importance of fully characterizing the behaviour of the ions, their interaction with the solvent and the electrode surface at the solid–liquid interface for the elucidation of the mechanism behind the increased capacitance. Nuclear magnetic resonance (NMR) is well suited to studying these systems because nuclear spins are exquisitely sensitive to their local environment. NMR is also nucleus-selective and can probe molecular motion in a range of dynamic regimes. Indeed, the interaction of molecules with porous carbon materials has been studied using NMR, both in working EDLC devices [13] , [14] , [15] , [16] , [17] , [18] and otherwise [19] , [20] , [21] , [22] , [23] , [24] , [25] , [26] , with nuclei close to the carbon surface being readily distinguished by their shift to lower frequencies (a shift to more negative p.p.m.). This characteristic shift of nuclear spins in strongly adsorbed (SA) or confined molecules/ions is a consequence of the shielding from the ring currents at the surface of the graphene-like sheets of carbon atoms, something that is well known in organic systems [27] , [28] , [29] , [30] , carbon nanotubes [31] and fullerenes [32] . As shown in recent work, the shift is nucleus-independent but does depend on the distance between the probe molecule and the carbon surface, and hence also depends on the sizes of the occupied pores [17] , [20] , [21] , [33] . This mechanism can lead to inhomogeneous line broadening of the SA peaks in the presence of large pore size distributions. Line broadening may also be caused by the local variations in susceptibility at the solid–liquid interface even when the pores are monodisperse, as is the case for molecules encapsulated in any porous media [34] , [35] . The diffusion and dynamics of the adsorbent molecules are crucial in this regard as they can average the variations in the local interactions over the time scales probed by NMR [20] , [21] . NMR is non-invasive and can be performed in situ on working EDLC devices [14] , [15] , [17] . Under these conditions, NMR has the potential to monitor the charge mechanism and follow the interactions and distributions of the anions and cations separately and in real time. This approach is more favourable than ex situ methods in which the disassembly of cells inevitably leads to physical and chemical changes taking place before measurements are taken. In situ NMR has been performed using modified cell designs to distinguish the effects at each electrode in separate experiments [14] , [15] , [17] . By contrast, here we present the first magnetic resonance imaging (MRI) experiments on EDLCs in situ on a working device of standard geometry (see Fig. 1e , Supplementary Fig. 1 and Supplementary Note 1 ). This procedure allows changes to be monitored in each element of the working EDLC cell simultaneously, unlike previous NMR experiments, which required separate experiments to measure the effects at each electrode [14] , [15] , [17] . Furthermore, we show that images can be collected in quick succession to capture snapshots of the system in non-equilibrium states during electrochemical cycling. This procedure allows changes in the cell to be monitored over time, giving evidence of a build-up of ions in their representative counter electrodes that lead to hysteresis effects in cyclic voltammetry (CV) experiments. The EDLC cell used is similar to commercially available systems, with activated carbon electrodes and an organic NEt 4 + /BF 4 − electrolyte solvated by acetonitrile. 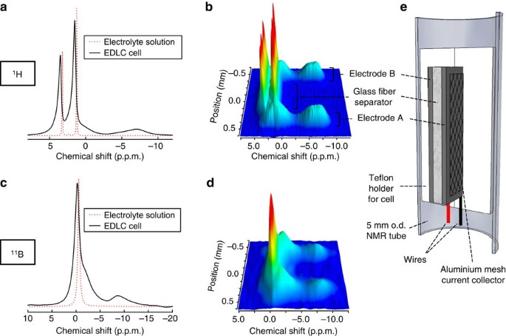Figure 1:1H and11B NMR spectra and CSIs of a pristine EDLC cell. (a)1H NMR spectra of the electrolyte alone (recycle delay, r.d.=10 s) and the EDLC cell (r.d.=4 s). (b)1H CSI of the EDLC cell with the components labelled (r.d.=0.1 s). (c)11B NMR spectra of the electrolyte (r.d.=10 s) and the EDLC cell (r.d.=3 s). (d)11B CSI of the EDLC cell (r.d.=3 s); (e) cross section through the cell design and illustration of component locations in the CSI. Figure 1: 1 H and 11 B NMR spectra and CSIs of a pristine EDLC cell. ( a ) 1 H NMR spectra of the electrolyte alone (recycle delay, r.d.=10 s) and the EDLC cell (r.d.=4 s). ( b ) 1 H CSI of the EDLC cell with the components labelled (r.d.=0.1 s). ( c ) 11 B NMR spectra of the electrolyte (r.d.=10 s) and the EDLC cell (r.d.=3 s). ( d ) 11 B CSI of the EDLC cell (r.d.=3 s); ( e ) cross section through the cell design and illustration of component locations in the CSI. Full size image NMR and chemical shift imaging of the EDLC cell The 1 H NMR signal from the pristine EDLC cell originates solely from the cation (NEt 4 + ), since the solvent (acetonitrile) is deuterated. Three sets of resonances are observed ( Fig. 1a ), corresponding to the -CH 3 and -CH 2 - groups in three distinct environments as has been described previously [14] , [15] : (i) free electrolyte in the separator, yielding the most intense and narrow peaks at shifts similar to those in the free electrolyte spectrum (1.3 p.p.m. for CH 3 and 3.3 p.p.m. for CH 2 ); (ii) a SA or confined environment close to the carbon surface that gives rise to the broad peaks shifted to low frequency (ca. −6.8 and −4.8 p.p.m. for CH 3 and CH 2 , respectively, 8.1 p.p.m. upfield from the corresponding free electrolyte peaks); (iii) a weakly adsorbed (WA) environment represented by peaks at similar shifts to those of the free electrolyte, but with significant broadening. The WA environment is either outside the pores or is in larger meso or macropores that are sufficiently large for there to be little or no chemical shift due to the larger distance of the ions away from the carbon surface and the associated ring current effects [15] , [33] . The electrode films do contain voids between the carbon particles and the polytetrafluoroethylene (PTFE) binder that can be expected to contain a sizeable volume of electrolyte, but since no free electrolyte peak is observed inside the electrodes in the chemical shift images (CSIs), this environment must give rise to at least part of the WA peak. Indeed, the WA peak is observed in all EDLC systems that use similarly constructed electrodes [14] , [17] , even when carbons with monodisperse nanopores are used [15] . The corresponding CSI, which gives spatially resolved chemical shift information ( Fig. 1b ), further substantiates these assignments, clearly showing that the SA and WA peaks are found only inside the electrodes, and emphasizing the distinction between the WA peaks and those of the free electrolyte. The 11 B spectrum and corresponding CSI ( Fig. 1c,d ) observe the anion (BF 4 − ), and show the same three environments as for the cation, demonstrating that in the pristine cell both ions occupy the same types of environment. 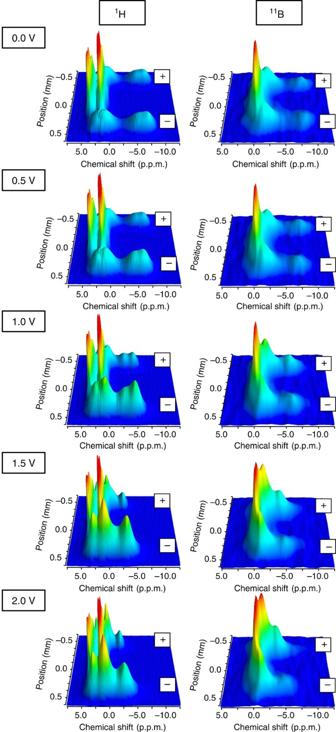Figure 2: CSIs acquired at equilibrated voltages. The1H (r.d.=0.1 s) and11B (r.d.=3 s) series were performed on separate cells. In situ constant voltage experiments Figure 2 shows 1 H and 11 B CSIs acquired in situ at constant voltages from 0 to 2 V. The images allow the behaviour of the ions in each electrode to be captured simultaneously. Slices extracted from these CSIs at positions corresponding to each electrode are displayed in Fig. 3 . It is clearly seen that the relative intensities of the 1 H signals are larger in the negative electrode, in line with a larger accumulation of cations, and the relative intensities of the 11 B signals are larger in the positive electrode, in line with a larger accumulation of anions there. The effects increase with voltage. A quantitative analysis of the intensities would likely be affected by charge-dependant relaxation losses [14] during the delay between signal excitation and detection. On the other hand, the voltage dependence of the chemical shifts and the line-broadening effects allow for a consistent analysis, as described below, which is compatible with the qualitative intensity changes mentioned here. Figure 2: CSIs acquired at equilibrated voltages. The 1 H (r.d.=0.1 s) and 11 B (r.d.=3 s) series were performed on separate cells. 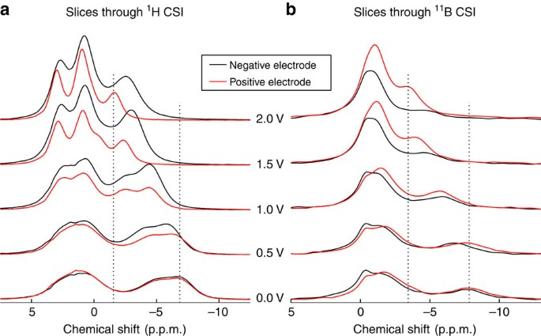Figure 3: Slices through the CSIs fromFig. 2corresponding to positions inside each electrode for (a)1H and (b)11B.  Full size image Figure 3: Slices through the CSIs from Fig. 2 corresponding to positions inside each electrode for ( a ) 1 H and ( b ) 11 B. Full size image On charging the cell to higher voltages, the SA peaks for both ions in both electrodes move to higher chemical shifts. This precludes the action of a shift mechanism dominated by the average ion surface distance, which would be both ion and electrode dependent. Instead, the shift can be primarily associated with the charge of the electrodes: the removal or addition of electrons into the electronic structure of the graphitic carbon sheets reduces the strength of the ring currents and therefore their de-shielding effects on local nuclei, as described recently by Wang et al. [14] , [17] Deconvolution of the slices in Fig. 3 yields a more detailed description of the charge dependence of the SA chemical shifts ( Fig. 4a,b ). The trends for the anions and cations are almost identical in each electrode, supporting the hypothesis that the changes in the chemical shifts are most strongly associated with the properties of the electrodes and not the ions. 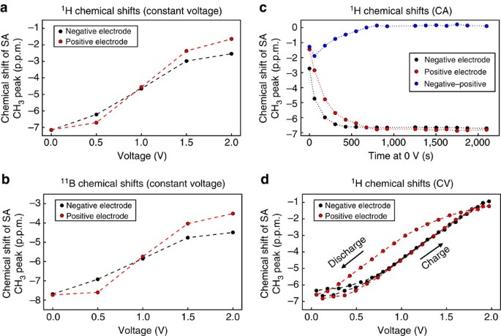Figure 4: Trends in the chemical shifts of the SA peaks during the constant voltage, CA and CV experiments. (a) The cation and (b) the anion held at constant voltages, (c) the cation during the equilibration period for a cell switched from +2 to 0 V in a CA experiment, and (d) during the 1st CV cycle of a pristine cell. For1H, the shift represents the peak corresponding to the SA CH3group. Figure 4: Trends in the chemical shifts of the SA peaks during the constant voltage, CA and CV experiments. ( a ) The cation and ( b ) the anion held at constant voltages, ( c ) the cation during the equilibration period for a cell switched from +2 to 0 V in a CA experiment, and ( d ) during the 1st CV cycle of a pristine cell. For 1 H, the shift represents the peak corresponding to the SA CH 3 group. Full size image There is a strong correlation between the upfield shift of the SA peaks during charging and a reduction in the linewidths of the SA and WA peaks (see Supplementary Fig. 2 and the associated description). This line narrowing occurs for the ions in both electrodes simultaneously. It is expected that the resonances for these environments are predominantly broadened by the microscopic magnetic field inhomogeneities at the interface between the surface of the carbon particles that are embedded in the electrode film, and the liquid-filled voids between them (the electrode films also contain a small amount of PTFE binder, which will have a slight influence on the effects discussed here but with no charge dependence). Importantly, the magnitude of the broadening is directly proportional to the difference between the susceptibilities of the solid and liquid media [36] , in this case between the carbon particles and the electrolyte solution inside the electrodes. On charging, electrons are added or removed from the electronic structure of the carbon, thereby changing its susceptibility, and therefore the linewidths of the SA and WA peaks. As for the effects on the SA chemical shifts, the trend in the line broadening is the same in the anode and cathode, confirming that the effects on the electronic structure of the carbon are similar whether electrons are added or removed from it. These effects establish a second method by which the electronic properties of the carbon can be probed in situ using magnetic resonance methods, although it would also be necessary to account for other intrinsic line-broadening mechanisms resulting from the dynamics of the ions within and between the pores and effects due to disorder in the carbon (resulting in distributions of pore sizes and electronic conductivities) [20] . This link between the EDLC charge and linewidths has not been established in previous NMR studies because the WA peaks in particular could not be fully resolved due to their overlap with the free electrolyte signal. In situ CV and chronoamperometry To explore the full capabilities of the MRI experiments, they were also applied to study the EDLC cell in non-equilibrium states. To this end, a chronoamperometry (CA) experiment was performed in which an EDLC cell equilibrated at +2 V was switched to 0 V and as the cell equilibrated, time-lapsed 1 H CSI experiments were used to monitor the cation SA peak’s chemical shift in real time ( Fig. 4c ). The results show the SA shifts of the cation in each electrode as they relax back to equilibrium in ~800 s. The observed behaviour is expected as the charge returns to being neutral on each electrode. More interestingly, however, the difference between the chemical shifts of the SA cations in each electrode show that initially there is a disproportionate decrease in the shift for the negative electrode compared with the positive. This difference (~1.9 p.p.m.) exceeds that observed at +2 V in this experiment (~1.3 p.p.m.) or in fixed voltage experiments in Fig. 4a (~0.9 p.p.m. ), suggesting that a non-equilibrium configuration of the system is being probed. It has been suggested based on NMR measurements [17] and calculations [37] that there are two distinct charge mechanisms taking place in EDLCs, type I dominating at low voltages (<0.75 V) and relying on ion rearrangements and the ejection of the co-ions from the electrodes, and type II contributing at higher voltages and describing counter-ion adsorption in the carbon pores. When the cell is equilibrated at +2 V, both electrodes are expected to have an excess of counter ions adsorbed in the carbon pores. As the cell starts to relax back to 0 V in the CA experiment, the type I and II mechanisms appear to act in reverse and there is a net ejection of the ions from the pores, while the adsorbed co- and counter-ions return to their equilibrium populations. The cations in the negative electrode are in excess in the carbon pores at the start of this process, and hence must be ejected during the relaxation (type I), while those that are adsorbed close to the carbon surface move further away from it on average (type II). The cations in the positive electrode move back into the pores (type I) as the anions migrate out, but can only return to their equilibrated average position inside the pores once the anions leave their adsorbed sites closest to the surface of the pore walls (type II). The average distances of the ions from the carbon surfaces are expected to influence the SA chemical shifts. Indeed, the large chemical shift difference between the SA shifts of the cations in the two electrodes correlates to them being disproportionally closer (compared with their equilibrium values in the constant voltage experiments) to the surface in the negative electrode as compared with the positive. This effect may suggest that the type I processes act more quickly during the equilibration to 0 V, which would also be compatible with these processes occurring at lower voltages on charge. Further NMR and MRI experiments are in progress to explore these phenomena in greater detail. To provide more evidence of the ion behaviour during charging, MRI experiments were performed on the cell under more realistic cycling conditions; in a CV experiment on a pristine cell. The 1 H CSIs from the CV experiment are shown in the Supplementary Movie in the Supplementary Information . The results mirror those from the constant voltage experiments, with the WA and SA peak shifts and line broadening correlating with the applied voltage. The deconvoluted chemical shifts of the SA peaks ( Fig. 4d ) show that on charge, the shifts of the cation SA peak behave almost identically in both electrodes. During discharge, however, a significant hysteresis develops in the chemical shifts of the cation SA peaks in the positive electrode: they become less shielded than at the equivalent voltages on charge, while there is no hysteresis for the cations in the negative electrode. The de-shielding corresponds to the ions being further away from the carbon surface on average than they were at the same voltages during charge. This corroborates the interpretation of the CA experiment as it suggests that the SA counter-ions are not completely removed from their adsorption sites inside the pores of the electrode and hence block the co-ions from returning to their equilibrium distribution. Thus, the type I mechanism must initially dominate during discharge because the counter ions that are SA in the type II mechanism during charge are not completely desorbed during discharge. There is precedent for a difference in the adsorption and charge storage behaviour of NEt 4 + and BF 4 − on carbon materials: Chmiola et al. [6] used the same NEt 4 + /BF 4 − electrolyte solution in EDLCs with a range of carbons with tuned pore sizes and observed that at almost all pore sizes, the positive electrode/anion combination registered the higher capacitance. The activated carbon used here has a range of pore sizes on the same scale as those investigated by Chmiola, and so may be expected to follow the same trend. In general, these properties may be related to the smaller ionic radius of BF 4 − (0.48 nm, unsolvated) compared with NEt 4 + (0.67 nm, unsolvated). The charge distribution in each molecule is also quite different, with the negative charge localized on the electronegative F atoms at the periphery of BF 4 − , whereas the positive charge in NEt 4 + is distributed over all of the H atoms in the molecule. This leads to increased screening in NEt 4 + , reducing the charge storage capacity on direct surface adsorption. The solvation energy of NEt 4 + compared with BF 4 − is also reduced, impacting charge storage mechanisms that involve a reversible stripping of the solvation shell [6] . It is interesting to note that commercial EDLC cells are typically pre-cycled to stabilise their electrochemistry before use. Our results, performed on a pristine cell, indicate that the changes occurring during the initial cycles may be a consequence of a build-up of the counter ions inside the pores (see also Supplementary Fig. 3 and associated discussion of cell aging). Understanding the material properties that influence this process may be a key step towards designing EDLCs with increased capacitances and power densities. In conclusion, in situ MRI methods have been presented and used to study EDLCs, allowing the simultaneous acquisition of chemical shift information from ions occupying each electrode in a working cell. By using 1 H and 11 B imaging, the anion and cation have been probed individually, giving detailed insight into the chemical shift mechanism for adsorbed environments in the carbon pores, and linking line-broadening effects to the electrode charges for the first time. Furthermore, it has been demonstrated that CSIs with high spectral and spatial resolution can be acquired fast enough to obtain snapshots of a working EDLC cell in real time during cycling, which has been used to distinguish the dominant charge storage mechanisms on charge versus discharge. These results can help guide future research efforts towards EDLCs with increased capacitance, while the methodology itself is novel and versatile, capable of providing unique insight into EDLCs and similar systems. Sample preparation EDLC electrodes were made from YP50F carbon (Kuraray Chemical) films. YP50F is an activated carbon with a microporous volume (<2 nm) of 70%, but it also contains mesopores (2–50 nm) and macropores (>50 nm) [38] . The 95% YP50F/5% PTFE films were prepared by heating YP50F carbon and a 60% PTFE dispersion in H 2 O (Aldrich) in ethanol for 1 h and were then rolled out to a film thickness of approximately 250 μm as described previously [14] . The films were cut to ~2 × 8 mm and dried under vacuum at 200 °C for 12 h before being placed in an argon glovebox. Symmetric EDLC plastic cells were assembled with electrodes of the same mass (2 mg for CV and 3 mg for constant voltage and CA) using a carbon-coated aluminium mesh as the current collector and a borosilicate separator (Whatmann type GF/B, thickness 0.68 mm). Note that a borosilicate separator was used instead of a thinner separator such as Celgard 2325, so as to increase the physical separation between the two electrodes, making the signals due to the two electrodes and electrolyte more readily resolvable. In total, 35 μl of 1.5 M NEt 4 + BF 4 − , tetraethylammonium tetrafluoroborate, (Fluka, electrochemical grade) in deuterated acetonitrile (99.96%, Aldrich) was added to the cell to ensure complete electrolyte saturation of the electrodes and the separator. The cell was then assembled and placed in a 5-mm NMR tube, as depicted in the schematic in Fig. 1e . A photograph of the cell is shown in Supplementary Fig. 4 . Cycling parameters CV experiments: the cell was cycled at a rate of 1 mV s −1 . Constant voltage experiments: the cells were held at voltages from 0.0 to 2.0 V in 0.5 V steps and the MRI experiments performed after the current reached an equilibrium state, or until d I /d t <1 μA s −1 . This equilibration typically took approximately 20 min, with a longer time required going from 1.5 to 2.0 V. CA experiments: the cell was equilibrated at 2.0 V and then switched to 0.0 V, with images collected during the equilibration period, approximately 35 min. MRI All MRI and NMR experiments were performed on a Bruker Ultrashield 9.4 T Avance I spectrometer containing a Bruker Micro2.5 gradient assembly and operating at 400.13 MHz for 1 H and 128.38 MHz for 11 B. A spin-echo chemical shift imaging (CSI) sequence was used to acquire the images, without slice selection. Before the CSI experiments, two-dimensional spin-echo images were used to align the cell with respect to the gradient axes. 1 H images were acquired using a Bruker Micro2.5 imaging probe with a 5 mm 1 H birdcage resonator. Excitation and refocusing pulses of 12.5 kHz nutation frequency were used with 64 phase-encoding steps incrementing the gradient strength between ±66 G cm −1 , giving a field of view of ~4.5 mm and nominal image resolution of 70 μm. The total echo time and repetition time were 670 μs and 100 ms, respectively. The 1 H chemical shift was referenced to the OH group in ethanol at 3.56 p.p.m. The 11 B images were acquired using a wide-band HR-50 probe (Cryomagnet Systems, Indianapolis) equipped with a 5-mm saddle coil. Radiofrequency pulses with 5 kHz nutation frequencies were used for excitation and refocusing. Experiments used 32 phase-encoding steps incrementing the gradient strength between ±57 G cm −1 , giving a field of view of ~4.5 mm and nominal resolution of 140 μm. The total echo time and repetition time were 1,160 μs and 3.0 s, respectively. The chemical shifts were referenced to 0.1 M boric acid solution at 19.6 p.p.m. NMR spectra were acquired using the same pulse powers as for the images, with relaxation delays as quoted with the results. How to cite this article: Ilott, A. J. et al. Multinuclear in situ magnetic resonance imaging of electrochemical double-layer capacitors. Nat. Commun. 5:4536 doi: 10.1038/ncomms5536 (2014).